Long-term projections and acclimatization scenarios of temperature-related mortality in Europe The steady increase in greenhouse gas concentrations is inducing a detectable rise in global temperatures. The sensitivity of human societies to warming temperatures is, however, a transcendental question not comprehensively addressed to date. Here we show the link between temperature, humidity and daily numbers of deaths in nearly 200 European regions, which are subsequently used to infer transient projections of mortality under state-of-the-art high-resolution greenhouse gas scenario simulations. Our analyses point to a change in the seasonality of mortality, with maximum monthly incidence progressively shifting from winter to summer. The results also show that the rise in heat-related mortality will start to completely compensate the reduction of deaths from cold during the second half of the century, amounting to an average drop in human lifespan of up 3–4 months in 2070–2100. Nevertheless, projections suggest that human lifespan might indeed increase if a substantial degree of adaptation to warm temperatures takes place. Scientists have described a wide range of potential negative impacts of climate change [1] on many vulnerable aspects of natural systems and human populations [2] , [3] , and particularly the sensitivity of our society to atmospheric temperatures [4] , [5] . In particular, increasing attention has been paid to warm extremes [6] , [7] , [8] , [9] , [10] , which are expected to become more frequent, longer and more severe [11] . Europe emerges as an especially responsive area to temperature rise, particularly during the warm season [12] . The record-breaking 2003 heat wave in western Europe has been described as an extremely unlikely event given the observed warming, and to share similar characteristics with future summers simulated by state-of-the-art climate models for the end of the 21st century [6] ( Fig. 1 ). Recent updates of summer heat-related mortality raise the initial estimates up to 70,000 excess deaths, of which 11,000 occurred in June, 10,000 in July, 15,000 during the first week of August and 24,000 during the second week [13] . However, the spatial distribution of the incidence was not homogeneous, with mortality excesses of 13.7% (22.9%), 11.8% (37%) and 11.6% (21.8%) during the summer (August) of 2003 in Spain, France and Italy, respectively [13] (cf. Fig. 1a,b with Supplementary Fig. S1 ). Figure 1: Comparison of summer 2003 temperature anomalies and scenario changes in summer mean conditions. Results for ( a , c , e ) daily mean and ( b , d , f ) apparent temperature (°C). Summer 2003 anomalies ( a , b ) were calculated as the difference between summer 2003 mean temperatures minus average summer temperatures for the 1998–2002 period. Scenario changes ( c , d ) were computed as the difference between multimodel mean projections for summers in 2090–2100 minus 1998–2008. ( e , f ) The difference between scenario changes minus summer 2003 anomalies. Full size image The risk of death under heat stress conditions is exacerbated in old people (impaired thermoregulation) living in urban areas (pollution, heat island effect) with pre-existing or chronic cardiovascular (heart attack, stroke) and respiratory diseases [4] , whereas exposure to cold can lead to direct effects such as hypothermia, or indirect pathologies such as cardiovascular disorders (hypertension, thrombosis) or respiratory infections (influenza, pneumonia) [14] . The incidence of these factors can be essentially reduced by means of physiological, behavioural and cultural adaptations of the society [4] , such as improvements in prevention, health care and early warning systems, the design of action plans for deprived people, a systematic vaccination against influenza, a change for healthier diets or a better acclimatization and insulation of buildings [1] , [5] , [15] , [16] . There is some evidence suggesting that these and other factors have already induced a reduction of mortality in some local areas [5] , [17] , [18] , but the potential of these strategies in each country varies greatly according to factors such as political decision making, technological development, profile demographics and underlying climatological conditions [4] . Under a hypothetical extremely severe warming scenario of +7 °C or more (for example, climate sensitivity has a 5% chance to exceed this value [19] ), heat stress would, however, start to impose a limit to human adaptability in some regions where metabolic heat dissipation would, for the first time, become impossible [20] . These constraints to human adaptability further stress the need for mitigation strategies contributing together with adaptation plans to tackle the problem of climate change [21] . These strategies, in turn, would ultimately maximize other cobenefits for health; for example, through improved air, water or food quality [22] , [23] , [24] . The present work describes the relationship between temperature, humidity and daily numbers of deaths in nearly 200 European regions representing more than 400 million people, and these links are then used to infer transient projections of mortality under greenhouse gas emission scenario simulations from eight state-of-the-art high-resolution climate models. For the first time, our study comprehensively addresses these relationships at the continental level and for the whole range of temperatures, showing a shift in the relative incidence of events in each tail. Results also indicate that the present climatology could be close to a state of minimum temperature-related mortality for Europe as a whole, mostly explained by the asymmetric relationship between temperature and mortality and the projected changes in the shape of the temperature distribution. Mortality projections are additionally computed according to innovative acclimatization scenarios, illustrating a hypothetical change in the vulnerability of the European society as a result of temperature rise. Dependency between temperature and mortality Daily temperatures [25] and numbers of deaths [13] corresponding to 187 NUTS2 regions (that is, second level of the Nomenclature of Territorial Units for Statistics [13] ) are studied here, which essentially correspond to the domain affected by the 2003 heat wave [6] , [8] and some neighbouring countries. Because of the extremely large differences in population between regions, they were grouped in 54 larger and more homogeneously populated areas. A transfer function (also referred here as temperature/mortality or T/M relationship) was estimated for the period with available observations (1998–2003), and used to convert simulated daily temperatures from other periods into daily mortality projections [15] , [26] , [27] . The transfer function is separately adjusted to data above (warm tail) and below (cold tail) the temperature of minimum mortality, or comfort temperature [15] . The fitting was assumed to be linear outside the range of observed temperatures as a conservative but reliable extrapolation of the T/M relationship. Further details regarding the methodology can be found in the Methods section. In the search of an optimal predictor of daily mortality, several variables based on temperature and/or humidity were tested. Figure 2 shows, for example, the relationship between daily mortality in Europe and daily maximum, mean ( T air ) and minimum temperature. The amount of variance linearly explained by these variables at daily resolution is relatively large, and of the same order of magnitude in all three cases ( r 2 =50% and 35–40% in the cold and warm tails, respectively). Note, however, that this fraction is clearly larger after applying a simple nonlinear transformation of daily temperatures (for example, variable T ′= a 0 + a 1 T + a 2 T 2 + a 3 T 3 explains r 2 =55% of daily mortality variance in the warm tail; see Methods ). Similar results are also found for daily mean apparent temperature ( T app ; Fig. 2b ), which accounts for the combined effect of temperature and humidity. This variable, widely used in the literature [28] , [29] , [30] , describes the body's ability to cool itself by evaporation and perspiration, especially during hot days [31] . For simplicity, only results corresponding to two of these variables are shown in this study. By default, apparent temperature is here used for the calculations, unless specified otherwise. At the same time, daily mean temperature is additionally used to provide alternative fittings and projections, in order to evaluate the sensitivity of results to the modulating role of decreasing summer humidity in the scenario simulations ( Supplementary Fig. S2 ). Figure 2: Observed relationship between daily temperatures and numbers of deaths in Europe. Dots depict the daily observed values of ( a ) mean, ( b ) apparent, ( c ) minimum and ( d ) maximum temperature (°C) and mortality (cases per million) for the 1998–2003 period. Pearson's correlations of daily data for days below or above the comfort temperature (dashed lines) are −0.7 ( a ), −0.7 ( b ), −0.71 ( c ) and −0.69 ( d ) for the cold tail, and 0.62 ( a ), 0.56 ( b ), 0.59 ( c ) and 0.61 ( d ) for the warm tail. Circles show the averages of data belonging to equally spaced intervals of temperature. Full size image The relationship between daily apparent temperature and mortality is further explored in Figure 3 ( Supplementary Fig. S3 for T air ). More detailed results by country can be found in Supplementary Figure S4 . The transfer functions display an asymmetric U-, V- or J-shape around the comfort temperature, as widely documented in the literature [4] , [14] , [15] , [32] ( Fig. 3a and Supplementary Fig. S3a ). The cold tail thus covers a larger range of temperatures, but the increase in mortality per unit of temperature is always much steeper in the warm tail (and especially in the case of T air ). In addition, the T/M dependency is usually nonlinear in the warm tail, whereas it is mostly linear in the cold tail (refer to ref. 4 for a schematic representation of these general properties). Note that comfort apparent temperatures range from 14 °C in central Europe to 25 °C in southern Spain, and they are significantly higher than annual mean apparent temperatures (between +3.5 and +12.5 °C, P <0.001 in a paired-sample t -test; Supplementary Fig. S5 ). Figure 3: Observed relationship between daily values and percentiles of apparent temperature and numbers of deaths in Europe. ( a ) Comfort temperature (purple circles; °C), and warm (red lines) and cold (blue) transfer functions (°C versus daily cases per million) for each area, as well as the average of the transfer functions for all 54 areas (black curve). Dashed straight lines correspond to the linear extrapolation of the T/M relationship inferred for events outside the range of observed temperatures. ( b ) Relationship between apparent temperature percentiles and daily mortality (cases per million), averaged for the 187 regions. To this aim, a percentile was assigned to each regional daily temperature, expressing its ordered position within the corresponding regional series (for example, the minimum/median/maximum value of a regional time series is assigned to percentile P0/P50/P100). Daily mortalities within each range of temperature percentiles were then averaged (circles and coloured horizontal thick lines). Full size image Regional daily temperatures were expressed as a percentile within the corresponding time series, and the relationship between daily temperature percentiles and mortality was then averaged for the set of 187 regions ( Fig. 3b for T app , Supplementary Fig. S3b for T air ). The warm tail appears to be restricted to the 3 summer months (also Fig. 4 below), and the cold tail thus covers a larger part of the year (that is, autumn, winter and spring). The increase in mortality per unit of temperature percentile is nearly the same above and below the comfortable part of the year (that is, around percentile P75). This increase becomes rapidly nonlinear during the warmest month of the year, and thus observed mortality is nearly the same for the set of the most extreme cold and warm temperature percentiles (that is, 30.2 cases per million for days below P1, and 29.8 cases per million for days above P99). Figure 4: Observations and projections of monthly temperature and mortality in Europe. ( a ) Monthly observed time series of daily mean temperature (black line; °C), apparent temperature (grey; °C) and total mortality (green; cases per million) for the 1998–2003 period, and averaged for the 54 areas. Red and blue lines and squares depict the evolution of monthly mortality maxima for the set of summer (June-July-August (JJA)) and winter (December-January-February (DJF)) months, respectively. The transfer functions inferred from daily mean and apparent temperature were then used to derive the projections of total mortality for the 1950–2100 period. ( b ) Maxima of monthly mortality projections for the set of summer (JJA, red and pink curves) and winter (DJF, dark and light blue) months, and inferred from daily mean (red and dark blue) and apparent (pink and light blue) temperature. Full size image Long-term projections of mortality Transfer functions describing the T/M relationship in the 54 European areas were used to infer future mortality projections by transforming simulations of daily temperature under A1B greenhouse gas emission scenario conditions [1] . Given the small scale of the defined areas, temperatures were obtained from eight state-of-the-art regional climate models providing transient simulations for the 1950–2100 period [33] . Future daily projections of deaths at the continental level were thus computed after summing the projection of mortality for each of the 54 areas. Further details are provided in the Methods section. Figure 4a depicts the observed monthly evolution of temperature and mortality in Europe. Both time series were strongly anticorrelated in 1998–2002, essentially because the monthly maximum of mortality in winter (955 monthly cases per million on average) was much larger than that in summer (765 monthly cases per million), compared with minima around June and September (730 monthly cases per million). Nevertheless, this seasonality in mortality radically changed in 2003, when differences between winter and summer monthly maxima became relatively small (915 and 860 monthly cases per million, respectively). More interestingly, mortality projections inferred from scenario simulations suggest that this shift in the structure of the seasonality could indeed represent a conservative glimpse of future conditions in summer ( Fig. 4b ). Temperature anomalies in summer 2003 were unprecedented in France, Switzerland and northern Italy (up to +5 °C in T app , +3.75 °C in T air ), but much less exceptional, for example, in northern and eastern Europe, the British Isles and most of the Iberian Peninsula (less than +2 °C; Fig. 1a,b ). Instead, mean summer A1B anomalies (and thus averaging all kinds of summers) for the end of the present century are expected to be higher than +3.25 °C (in T app ) or +2.5 °C ( T air ) in continental Europe, and to exceed +4 °C (in T app ) or +3.5 °C ( T air ) in the entire Mediterranean area ( Fig. 1c,d ). As a result, the abnormal summer of 2003 only exhibited slightly warmer temperatures in the core of the hot spot (that is, some local areas in France, Switzerland and northern Italy), compared with future climatologically normal summers simulated for the end of the century (thick contours in Fig. 1e,f ). Note that future daily heat wave anomalies will in turn mount on these warmer underlying summer conditions [34] . When averaged for the European domain, and assuming unchanged transfer functions (that is, scenario with no adaptation) and profile demographics (for example, same population size and age), mortality projections for monthly maxima in summer are therefore expected to be clearly larger than that in summer 2003, steadily rising up to 900 (when inferred from T app ) or 970 ( T air ) monthly cases per million in 2091–2100 (pink and red curves in Fig. 4b , respectively). Instead, the monthly mortality peak in winter will slowly decrease in both cases down to 860 monthly cases per million in 2091–2100 (overlapped blue curves in Fig. 4b ), and thus monthly maxima in both seasons are estimated to be of the same magnitude around 2080 ( T app ) or 2050 ( T air ). More detailed projections of mortality at the continental level are provided in Figure 5 and Supplementary Figure S6 . Despite the reversal in the bimodal structure of mortality, which did not occur in 2003, cold-related deaths (solid blue line in Fig. 5a,b ) will still represent the major factor contributing to total mortality, compared with the relatively lower incidence of heat effects (solid red curve in Fig. 5c,d ). Assuming again unchanged transfer functions and profile demographics, the rise in heat-related mortality will nearly (completely) compensate for the decrease in cold-related deaths during the first two-thirds (the last third) of the century (solid green line in Fig. 5e,f ). Total mortality will thus keep decreasing at a nearly constant rate until 2025–2055, but then the number of deaths will start to monotonically rise, with a final net increase in overall mortality of up to +15,000 annual deaths in 2070–2100 (that is, a drop of about 3–4 months in human lifespan). Note that the initial reduction in total mortality would not occur if the effect of decreasing summer humidity was suppressed, with mortality estimates rising up to +50,000 annual cases at the end of the century (that is, almost a year in human lifespan; solid green curve in Supplementary Fig. S6e,f ). Figure 5: Projections of mortality according to scenarios of adaptation to warm and/or cold apparent temperatures. Annual mean values of mortality (million cases) for rolling 31-year periods were summed at the continental level for the 54 areas. ( a , c , e ) Mortality projections for a scenario with only decreased susceptibility to warm temperatures ( g ). For b , d , f , increased susceptibility to cold temperatures is also assumed ( h ). Solid lines in the projections correspond to a scenario with no adaptation (that is, R =0), and dashed curves indicate that the warm and/or cold transfer functions are shifted by R ·Δ μ degrees in the temperature space (0< R ≤1), where Δ μ represents the time-varying increase in annual mean apparent temperatures relative to 1980–2010. Horizontal black lines depict the annual mean mortality for this reference period. Blue, red and green colours correspond to projections of mortality computed for days within the cold tail, the warm tail and the whole range of temperatures, respectively. Note that the threshold dividing the range of temperatures into the warm and cold tails was here shifted by R ·Δ μ /2 and R ·Δ μ degrees in g and h , respectively. Coefficient R is here shown for values 0.0 (darker line), 0.1, 0.2,..., 0.9, 1.0 (lighter curve). Full size image These changes in continental mortality are not, however, representative of the 54 European areas ( Supplementary Fig. S7 ). If the role of summer humidity was not taken into account, total mortality at the end of the century would rise in most of the southern areas, and decrease only in England/Wales and Denmark ( Supplementary Fig. S7a ). However, when this effect is accounted, the real magnitude of projected changes is somewhat smaller ( Supplementary Fig. S7b ). More interestingly, differences between both cases are larger in the Mediterranean countries, where humidity is expected to substantially decrease ( Supplementary Fig. S2 ). Nevertheless, projections of European mortality cannot be simply explained by a shift in annual mean temperatures alone ( Fig. 6 and Supplementary Fig. S8 ). Considering the original set of transfer functions inferred from observations, and assuming again unchanged profile demographics, a minimum in European mortality would thus occur if temperatures were simply +3.8 °C (in the case of T app ; Fig. 6a ) or +2.6 °C ( T air ; Supplementary Fig. S8a ) warmer than in 1998–2003, with no other changes in the probability distribution function (PDF) of temperature (that is, only annual mean temperatures are shifted). This temperature anomaly is indeed expected to occur in the simulation ensemble around 2080–2110 (in the case of T app , when temperature projections are linearly extrapolated from 2100 onwards; blue line in Fig. 6b ) or 2061–2091 ( T air ; Supplementary Fig. S8b ), and thus also the minimum in mortality if only annual mean temperatures were changing. 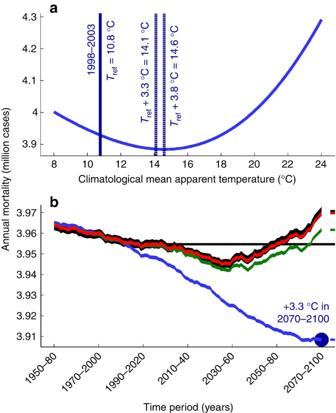Figure 6: Projections of total mortality inferred from scenario changes in only the mean, standard deviation and/or skewness of apparent temperatures. Annual mean values of mortality (million cases) for rolling 31-year periods were summed at the continental level for the 54 areas. (a) Projections of mortality inferred from observed daily temperatures and observed transfer functions (1998–2003). In this case, however, the climatological mean of each temperature time serieswas retuned throughout the domain of temperaturesand annual projections of mortality were then recomputed and expressed as a function of the new climatological mean(b) Multimodel mean projections of mortality inferred from simulated daily temperatures (1950–2100) and observed transfer functions (1998–2003). Simulated temperature time series for the 1980–2010 period are here retuned according to multimodel mean scenario changes in the mean (M-A1B, blue curve), the mean and standard deviation (MS-A1B, green), or the mean, standard deviation and skewness (MSW-A1B, red) of the temperature PDF, and projections of mortality are then compared with those directly inferred from the transient simulations (A1B, black). The horizontal black line depicts the annual mean mortality for the reference period 1980–2010. Figure 6: Projections of total mortality inferred from scenario changes in only the mean, standard deviation and/or skewness of apparent temperatures. Annual mean values of mortality (million cases) for rolling 31-year periods were summed at the continental level for the 54 areas. ( a ) Projections of mortality inferred from observed daily temperatures and observed transfer functions (1998–2003). In this case, however, the climatological mean of each temperature time series was retuned throughout the domain of temperatures and annual projections of mortality were then recomputed and expressed as a function of the new climatological mean ( b ) Multimodel mean projections of mortality inferred from simulated daily temperatures (1950–2100) and observed transfer functions (1998–2003). Simulated temperature time series for the 1980–2010 period are here retuned according to multimodel mean scenario changes in the mean (M-A1B, blue curve), the mean and standard deviation (MS-A1B, green), or the mean, standard deviation and skewness (MSW-A1B, red) of the temperature PDF, and projections of mortality are then compared with those directly inferred from the transient simulations (A1B, black). The horizontal black line depicts the annual mean mortality for the reference period 1980–2010. Full size image Instead, changes in the shape of the temperature PDF, and not only in the annual mean, explain the projected changes in European mortality shown in Figure 5 and Supplementary Figure S6. Ballester et al . [35] stated that mortality projections inferred from simulated temperature time series can be successfully reproduced after transforming the present temperature PDF according to simulated scenario changes in only the mean, standard deviation and skewness of the temperature PDF (MSW-A1B in Supplementary Fig. S9 ), with no other information from future simulated temperature time series (for example, changes in the properties of future extremes). This hypothesis is validated here, in the sense that this simple methodology provides virtually equal projections of mortality (red lines in Fig. 6b and Supplementary Fig. S8b ) than those inferred from the simulations themselves (black curves). Note, however, that when the skewness is maintained constant, and thus simulated changes in the asymmetry of the PDF are not taken into account (MS-A1B in Supplementary Fig. S9 ), mortality is slightly underestimated (green lines in Fig. 6b and Supplementary Fig. S8b ). Scenarios of acclimatization to warmer conditions Given the general lack of knowledge about future adaptation scenarios, all these results are inferred from a future hypothetical warmer world with unchanged vulnerability of the European society to warm and cold temperatures. Contrary to this assumption, some authors have stressed the time-varying structure of the T/M dependency [15] , [17] . For instance, McMichael et al . [4] proposed a conceptual framework with decreased mortality rates in the warm tail. As temperatures rise, warm days will become more frequent, and the society might therefore (spontaneously or not) adapt to some extent to the new environmental conditions in summer. This conceptual model is here studied by shifting the comfort temperature by R ·Δ μ /2 degrees and the warm transfer function by R ·Δ μ degrees, where R is a constant factor ranging from 0 to 1, and Δ μ represents the time-varying increase in annual mean temperatures relative to 1980–2010 ( Fig. 5g ). At the same time, the society might also lose some degree of acclimatization to cold conditions, as a result of the decrease in the frequency of these events, and thus results were also calculated for a scenario in which the comfort temperature and both transfer functions are shifted by R ·Δ μ degrees ( Fig. 5h ). Both scenarios are here exposed in order to explore a large range of mortality projections inferred from the still highly uncertain response of the society to temperature rise. For simplicity, results corresponding to a different degree of adaptation in each tail (that is, 0< R cold < R warm ≤1) are not shown here, but they can be simply inferred from the two particular cases in Figure 5g (0= R cold ≤ R warm ≤1) and h (0≤ R cold = R warm ≤1). Note that these acclimatization scenarios refer only to those modifications in the T/M relationship that are associated with warming environmental conditions. These changes therefore exclude those that might equally occur in a naturally fluctuating scenario with no anthropogenic climate trends; for example, a general rise in human lifespan due to continuous improvements in health care systems and treatments, or the increase in the susceptibility to extreme temperatures as a result of population ageing in developed societies such as Europe [36] . Factor R here represents the acclimatization pace of the society to warming environmental conditions, with R =0 ( R =1) defining a scenario of no acclimatization (immediate gain and/or loss of acclimatization to warm and/or cold temperatures, respectively). Up to our knowledge, the real value of this coefficient has never been estimated in the literature, as observed temperature trends have been small compared with future projections. Unless strict adaptation strategies are specifically implemented, we should expect a scenario with rather small values of R . Otherwise, vulnerability of human beings to a temperature event would be essentially connected with its relative occurrence (that is, the larger the frequency, the lower the vulnerability), and then the difference between comfort and annual mean temperatures would be small in the present climate (contrary to results in Supplementary Fig. S5 ). In addition, we expect that coefficient R warm decreases in parallel with temperature rise, as human adaptability is subject to nonlinearities and limits imposed by heat stress [20] . Despite these considerations, the degree of adaptation of societies to warmer climate conditions is an issue subject to huge uncertainties [4] , and this general lack of knowledge is here solved by exploring the whole range of scenarios providing hypothetical acclimatization pace levels. The increase (decrease) in heat (cold)-related mortality is projected to be substantially lower in some of these acclimatization scenarios ( Fig. 5a–d ). Note that differences between projections of heat-related mortality (cf. Fig. 5c,d ) do not reflect a change in adaptation to warm temperatures, but only the sensitivity of results to the choice of the new comfort temperature (cf. Fig. 5g,h ). More interestingly, even if the shift to warmer values of the transfer function in both tails was assumed to be equal to that of the temperature PDF mean (that is, R =1 in Fig. 5h ), heat (cold)-related mortality would still be projected to increase (decrease), showing the combined effect of changes in the shape of the PDF and the asymmetry in the T/M relationship. In this case, the rise in heat-related deaths (up to +110,000 annual cases in 2070–2100; lighter curve in Fig. 5d ) would not be completely compensated by an equivalent decrease in the cold tail (–71,000 annual deaths; Fig. 5b ), with a net increase in overall mortality of up to +39,000 annual cases in 2070–2100 (that is, a drop of about 8–9 months in human lifespan; Fig. 5f ). Changes in total mortality would also be sensitive to a hypothetical loss of acclimatization to cold temperatures (cf. Fig. 5e,f ). Although sensitivity is low for relatively small values of R, there is actually room for a substantial reduction in total mortality in a scenario with large adaptation to warm days and unchanged susceptibility to cold temperatures, with a net reduction in overall mortality of up to −78,000 annual deaths in 2070–2100 (that is, a rise of around a year and a half in human lifespan; Fig. 5e ). In the more developed countries, the population aged 60 years or above is increasing at the fastest pace ever (+1.9% annually), and it is expected to increase by more than 50% until 2050 (ref. 36 ). In particular, Europe has, at present, the oldest population worldwide, with a median age of nearly 40 years, and it is expected to reach 47 years in 2050 (ref. 36 ). Around 60% of the people who died in France were aged 75 or above during the 2003 heat wave [37] , and the risk of this kind of episodes has been at least doubled simply as a result of temperature rise [38] . Indeed, the IPCC AR4 states with very high confidence that climate change contributes to the global burden of disease and to increased mortality [5] , and particularly that the higher frequency of heat waves and the excess deaths associated with the European 2003 event are likely to be linked to climate change [1] . These and other factors such as the increasing urban population [39] , taken together, provide a glimpse into future summer conditions that the European society will have to face once mean temperatures start to speed up. Our analyses point to a change in the seasonality of mortality, with maximum monthly incidence progressively shifting from winter to summer. Results also indicate that the present climatology could be close to a state of minimum temperature-related mortality for Europe as a whole, even though projection trends of mortality are small in relative terms and different for northern and southern Europe. Indeed, even assuming unchanged profile demographics and taking into account the modulating role of decreasing summer humidity, the total number of deaths would start to monotonically increase around the middle of the 21st century, amounting to an average drop in human lifespan of up to 3–4 months in 2070–2100. This conclusion contradicts previous assertions suggesting that increases in heat-related mortality will be overweighed by larger declines in cold-related mortality, given that annual mean temperatures are expected to become more comfortable in terms of mortality. Instead, two factors with opposite contribution explain this non-trivial evolution of mortality incidence in the context of climate change. On the one hand, the decreasing difference between comfort and annual mean temperatures is expected to increase the number of comfortable days. On the other hand, the asymmetric shape of the transfer functions defines a scenario in which mortality rise due to the set of new warm days will compensate the decline in deaths as a result of the lower occurrence of cold days. The contribution of new warm days will be even larger given the expected flattening and shift to positive skews of the temperature PDF in the whole domain (that is, rise in standard deviation and skewness, respectively; see scenario anomalies in ref. 35 ). These changes will ultimately lead to an increase in the frequency of warm extremes and a decrease in the number of comfortable days. The trend reversal in temperature-related mortality before the middle of the century after several decades of decreasing rates suggests that the European society will have to take clear steps to deal with a new reality in the medium and long term. Whether this adaptation will occur spontaneously or will require planned strategies is a non-trivial question that is far beyond the scope of the present work. As an example, the French authorities implemented new plans including warning systems, health surveillance and structural improvements to residential institutions just after the 2003 episode [40] , [41] . Our results indeed suggest that total mortality at the end of the century might largely decrease if the society rapidly adapts to the effects of warm temperatures, amounting to an increase of up to a year and a half in human lifespan in the most optimistic, albeit quite unrealistic, of the acclimatization scenarios. This result stresses the importance of adaptation and mitigation strategies that need to be developed in order to prepare the European societies for projected temperatures for the second half of the century. Mortality data Daily regional counts of mortality from 1 January 1998 to 31 December 2005 were collected for 16 European countries representing around 405 million people. These countries are Austria, Belgium, Croatia, the Czech Republic, Denmark, France, Germany, Italy, Luxembourg, Netherlands, Poland, Portugal, Slovenia, Spain, Switzerland and the United Kingdom (England and Wales only). In some regions, however, records were only available until the end of 2003 or 2004, and therefore results at the continental level are only shown for the common period 1998–2003 (ref. 13 ). Temperature data Daily high-resolution observations (0.25°×0.25°) and A1B greenhouse gas emission scenario simulations (25×25 km 2 ) of daily maximum, mean, minimum and dew point ( T dewpt ) temperature were derived from the ENSEMBLES project [33] . Daily mean apparent temperature was calculated according to with all variables expressed in °C (refs 28 , 29 , 30 , 31 ). Only regional climate models with transient simulations expanding from 1950 to 2100 were taken into account in the analysis, namely C4I:RCA3 (driven by HadCM3Q16), CNRM:Aladin (ARPEGE-RM5.1), DMI:HIRHAM5 (ECHAM5-r3), ETHZ:CLM (HadCM3Q0), ICTP:RegCM3 (ECHAM5-r3), KNMI:RACMO2 (ECHAM5-r3), MPI:REMO (ECHAM5-r3) and SMHI:RCA (ECHAM5-r3). Regional analysis Population estimates at the regional level were provided by Eurostat for the year 2003. Because of the extremely large differences in population between regions (from 18 million in North Rhine-Westphalia to <100,000 in some Slovenian regions), regions were grouped in 54 larger and more homogeneously populated areas ( Supplementary Fig. S5 ). Several factors were taken into account in this process, such as geographical proximity, state borders (for example, similar warning systems or adaptation measures might be applied in each country) and similarities in regional T/M dependencies or comfort temperatures. Projections of mortality at the continental level were, however, unaffected by the way of grouping regions (results not shown). Definition of the transfer functions The T/M dependency in a region, area or country was estimated as follows. The range of observed temperatures was divided into equally spaced intervals [15] , [17] , [20] . Days belonging to each interval were grouped and daily temperature and mortality data within each interval averaged (circles in Supplementary Fig. S4 ). Interval mean mortality was smoothed by means of a centred 31-term filter, corresponding to nearly 3 °C intervals [15] , [17] , [42] , and the lowest value defined the interval of comfort temperature [4] , [42] . This threshold divides the range of temperatures into the warm and cold tails (red and blue colours in Supplementary Fig. S4 ). Given the nonlinear dependency between temperature and mortality [4] , [31] , [32] , especially for the most extreme warm temperatures [20] , the T/M relationship was defined as a polynomial of order 3. For each tail of a given area, the optimal coefficients { a 0 , a 1 , a 2 , a 3 } from were found by means of a least squares fitting of interval mean temperature and mortality data. Alternative transfer functions Alternative functions for the fitting of daily temperature and mortality data were tested, such as a simple linear approach but the amount of explained variance was considerably lower (for example, Fig. 2 ). The only alternative function explaining an equivalent amount of variance was the exponential fitting but it was not used in this study because it would require a case-by-case supervision of coefficients { c 0 , c 1 , c 2 , c 3 , c 4 } in each area, in order to avoid unrealistically large slopes of the transfer function for the warmest temperatures (results not shown). In any case, the sensitivity of projections to the choice of the function can be considered relatively small, and the chosen fitting a compromise between the different options ( Supplementary Fig. S10 ). Linear extrapolation of the T/M relationship Extrapolated mortality outside the range of observed temperatures was here assumed to increase linearly (dashed straight lines in Supplementary Fig. S4 ). Note that this assumption might lead to an underestimation of heat-related mortality in a future warmer climate. The effect of this choice was, however, rather small ( Supplementary Fig. S11 ), due to the relatively very small number of days outside the range of observed temperatures, even in a strongly warmed climate. The linear extrapolation was, however, applied in order to derive a conservative but reliable estimation of the expected heat-related mortality increase due to temperature rise. How to cite this article: Ballester, J. et al . Long-term projections and acclimatization scenarios of temperature-related mortality in Europe. Nat. Commun. 2:358 doi: 10.1038/ncomms1360 (2011).